Inferred time- and temperature-dependent cation ordering in natural titanomagnetites Despite years of efforts to quantify cation distribution as a function of composition in the magnetite–ulvöspinel solid solution, important uncertainties remain about the dependence of cation ordering on temperature and cooling rate. Here we demonstrate that Curie temperature in a set of natural titanomagnetites (with some Mg and Al substitution) is strongly influenced by prior thermal history at temperatures just above or below Curie temperature. Annealing for 10 −1 to 10 3 h at 350–400 °C produces large and reversible changes in Curie temperature (up to 150 °C). By ruling out oxidation/reduction and compositional unmixing, we infer that the variation in Curie temperature arises from cation reordering, and Mössbauer spectroscopy supports this interpretation. Curie temperature is therefore an inaccurate proxy for composition in many natural titanomagnetites, but the cation reordering process may provide a means of constraining thermal histories of titanomagnetite-bearing rocks. Further, our theoretical understanding of thermoremanence requires fundamental revision when Curie temperature is itself a function of thermal history. The most important natural magnetic materials are the titanomagnetites, Fe 3− x Ti x O 4 with endmembers magnetite ( x =0) and ulvöspinel ( x =1). Ferrimagnetism in these materials arises from an antiferromagnetic coupling of the A and B sublattices of the inverse spinel structure, with a net spontaneous magnetization that is determined by the proportions and the valence states of the magnetic cations in the A (tetrahedral) and B (octahedral) sites [1] , [2] , [3] , [4] , [5] , [6] , [7] , [8] , [9] , [10] , [11] , [12] . The Curie temperature ( T C ) is directly related to the strength of the exchange interactions within and especially between the sublattices, which in turn depend on the site occupancy of the magnetic cations [13] , [14] , [15] . The ideal structural formulas of the endmembers magnetite and ulvöspinel are Fe 3+ [Fe 3+ Fe 2+ ]O 4 and Fe 2+ [Fe 2+ Ti 4+ ]O 4 , respectively, where the square brackets indicate cations in octahedrally coordinated (B) sites and unbracketed cations are in tetrahedrally coordinated (A) sites. Magnetite is a so-called 2-3 spinel (one divalent and two trivalent cations per formula unit), while ulvöspinel is a 4-2 spinel. Both are inverse, meaning that the trivalent ions are equally divided among the A and B sites in magnetite, and the divalent ions likewise partitioned in ulvöspinel [16] . In spinels generally, the actual cation distribution varies with temperature, and ideal ordered distributions, with perfect segregation of cations onto the A and B sites, are only achieved as T approaches 0 K (for example, refs 16 , 17 ). With randomizing thermal energy the cations can, to varying extents, exchange between tetrahedral and octahedral coordination, resulting in an imperfectly ordered distribution that is increasingly randomized at higher temperatures [17] , [18] . Intermediate composition titanomagnetites (0< x <1) are complex spinels, with three different metal cations and valence states (Fe 2+ , Fe 3+ and Ti 4+ ), and significant work has been done with synthetic samples to deduce the degree, form and temperature dependence of cation order and to understand its effects on fundamental magnetic properties [1] , [2] , [3] , [4] , [5] , [6] , [7] , [8] , [9] , [12] , [19] , [20] , [21] , [22] . In natural titanomagnetites, additional complexity is added by the common presence of substituted cations (for example, Al, Mg and Mn) and variable degrees of cation deficiency, and we are unaware of any previous studies linking changes in fundamental properties such as T C to reordering of the cation distribution in natural titanomagnetites. Our ability to address these issues experimentally depends upon the temperature dependence of the ordering/disordering rate, which is more rapid at higher temperatures. For example, in the inverse spinel magnesioferrite (Fe 3+ [Fe 3+ Mg 2+ ]O 4 ), the well-documented kinetics of cation reordering are slow enough at temperatures below ~450 °C that a low degree of order achieved at elevated temperatures can be ‘quenched in’ if the sample is rapidly cooled [14] . In contrast, many careful experiments have shown that the kinetics of cation ordering in stoichiometric titanomagnetites are too rapid to preserve the relatively disordered states characteristic of high temperatures on cooling to room temperature [3] , [8] , [12] . This is thought to arise from a combination of a strong octahedral site preference for Ti 4+ at all temperatures [12] , [23] and rapid reordering of the remaining Fe 2+ and Fe 3+ via electron hopping [4] . A notable exception is the work of Lattard et al . [15] , in which cation reordering is invoked to explain irreversible thermomagnetic behaviour in synthetic cation-deficient titanomagnetites of intermediate composition ( T C measured on warming < T C measured on cooling by ≤40 °C). We show here for the first time experimental results documenting very large and systematic changes in T C in natural titanomagnetites, resulting from laboratory thermomagnetic measurements and isothermal annealing at moderate (350–400 °C) temperatures, and we interpret the results in terms of time- and temperature-dependent cation distributions. Oxide composition Samples used in this study are dacitic pumice or ash from the 1980 eruption at Mt St Helens (MSH) and the 1912 Novarupta (NV) eruption in Alaska. Like most natural titanomagnetites, the homogeneous grains present in these rocks have moderate degrees of Mg and Al substitution ( Fig. 1 and Supplementary Table S1 ) and minor amounts of Mn. Average compositions for MSH and NV are, respectively, Fe 2+ 1.20 Fe 3+ 1.31 Ti 0.30 Mg 0.09 Al 0.09 Mn 0.01 0 4 and Fe 2+ 1.17 Fe 3+ 1.40 Ti 0.26 Mg 0.06 Al 0.08 Mn 0.03 0 4 . The composition of these titanomagnetites overlaps data from most andesites, dacites and rhyolites [24] , as well as some basalts [25] . Most samples additionally contain a variable fraction of oxyexsolved titanomagnetites. 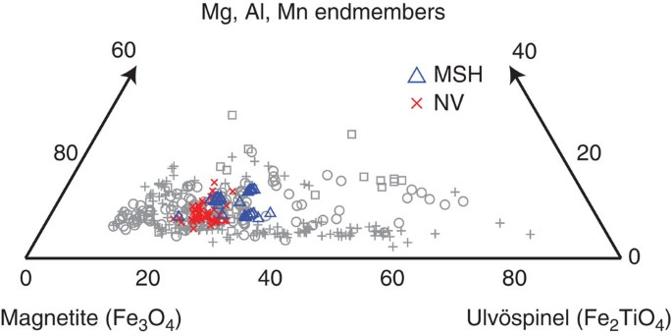Figure 1: Cubic oxide endmember compositions. MSH, blue triangle; NV, red × . Grey symbols from compilation of Ghiorso and Evans24; cross, rhyolite; circle, dacite; and square, andesite. Figure 1: Cubic oxide endmember compositions. MSH, blue triangle; NV, red × . Grey symbols from compilation of Ghiorso and Evans [24] ; cross, rhyolite; circle, dacite; and square, andesite. Full size image Thermomagnetic behaviour of samples in natural state The hallmark thermomagnetic behaviour of many of these samples in their natural state (before annealing) is a distinct form of irreversibility ( Fig. 2 ). During stepwise, multicycle measurement of susceptibility versus temperature ( χ ( T ); see Methods), we observe reversible χ ( T ) for cycles with T max up to ~400 °C; these cycles do not reach the T C , which exceeds 400 °C for most samples during initial heating. Usually, the first cycle in which T max exceeds 400 °C or 450 °C passes through T C and is strongly irreversible; T C for the cooling curve is significantly lower than that for the heating curve. In most cases subsequent heating/cooling cycles are reversible, but in some cases (for example, Fig. 2a ) there is a second irreversible cycle that causes an additional decrease in T C . For all samples, T C reaches a relatively stable value of ~345–375 °C for cycles with T max ≥500 °C, and we interpret this T C to be associated with the homogeneous titanomagnetite grains. For samples containing a significant population of oxyexsolved grains, a second T C is observed above 550 °C and is unaffected by cycling to higher temperatures ( Fig. 2c ). Typically there is little to no change in room-temperature susceptibility, despite the large changes in T C . Identical behaviour is observed under heating in air or in argon, as well as during temperature-dependent measurements of saturation magnetization ( M S ) in helium. 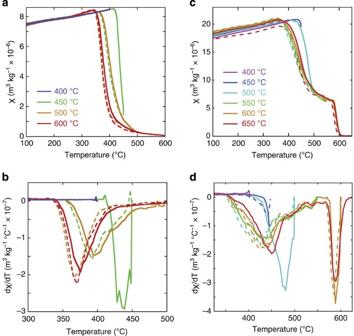Figure 2: Susceptibility measurements during stepwise heating of previously unheated samples. Samples (a) MSH008-D and (c) NV17-A, starting from the natural state. Solid and dashed lines, respectively, indicate measurement on heating and cooling, and colour shading represents the maximum temperature achieved during each heating cycle. (b,d) First-derivative curves, using three-point moving average. Note that horizontal axis scaling is different than inaandc. MSH008-D contains only homogeneous titanomagnetite withTC<450 °C. NV17-A contains two populations of Fe-Ti oxides: oxyexsolved grains with ilmenite lamellae in magnetite (TC~580 °C); and homogeneous titanomagnetites (TC<500 °C) for which the Curie temperature changes during the experiment. Figure 2: Susceptibility measurements during stepwise heating of previously unheated samples. Samples ( a ) MSH008-D and ( c ) NV17-A, starting from the natural state. Solid and dashed lines, respectively, indicate measurement on heating and cooling, and colour shading represents the maximum temperature achieved during each heating cycle. ( b , d ) First-derivative curves, using three-point moving average. Note that horizontal axis scaling is different than in a and c . MSH008-D contains only homogeneous titanomagnetite with T C <450 °C. NV17-A contains two populations of Fe-Ti oxides: oxyexsolved grains with ilmenite lamellae in magnetite ( T C ~580 °C); and homogeneous titanomagnetites ( T C <500 °C) for which the Curie temperature changes during the experiment. Full size image Thermomagnetic behaviour of annealed samples We selected samples ( Supplementary Table S2 ) from four different locations at both MSH and NV on which to conduct detailed annealing experiments. In the isothermal annealing experiments, individual specimens were heated in air for times ranging from 10 −1 to 10 3 h at 350 and 400 °C. These temperatures are below the cation ordering closure temperature for the system, as will be further explained below. After the scheduled exposure time, specimens were removed from the furnace and allowed to cool in air, achieving room temperature in <10 min. Following each anneal, we measured susceptibility on warming and cooling in air at a rate of 10 °C min −1 from 25 °C to a T max of 600 °C or 650 °C, after which the specimens were placed back in the furnace for the next annealing treatment. Supplementary Table S3 documents the order of treatments for each specimen. The decrease in T C during the thermomagnetic experiments ( Fig. 2 ) is fully ‘reversible,’ in the sense that T C can be increased again by isothermal annealing at moderate temperatures. Results from specimen MSH002-G-5 ( Fig. 3a ) are representative and demonstrate that T C measured on heating varies strongly with anneal time, increasing by >100 °C after annealing for 144 h at 350 °C. By contrast, T C measured on cooling from 600 °C is extremely consistent at T C ~345 °C for this specimen, regardless of any prior heat treatment ( Fig. 3a ). There is a single dominant T C on the heating branch after each treatment, indicating that the process responsible for the increase in T C occurs progressively and homogeneously throughout the entire volume of the titanomagnetites. Similar results were found for homogeneous titanomagnetites in specimens that also contain a population of oxyexsolved grains ( Fig. 3c ). The oxyexsolved grains have a (comparatively) reversible susceptibility with T C ~585 °C, regardless of annealing. We do note that with repeated annealing and thermomagnetic measurements, several samples tended to undergo what we interpret to be slight but progressive irreversible oxidation. This is reflected in the slight but progressive (in time) decrease in the proportion of the low- T C phase in the cooling curves, as can barely be discerned in Fig. 3c . 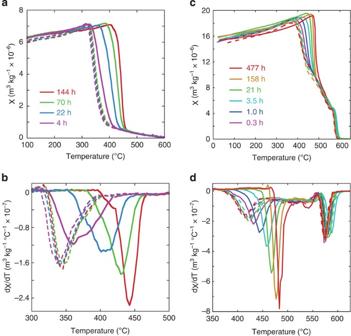Figure 3: Curie temperature variation with anneal time. (a) Temperature-dependent susceptibility measurements and (b) derivative curves from samples MSH002-G following annealing at 350 °C for different durations. (c,d) Same data for NV39-A following annealing at 400 °C for different durations. Solid and dashed lines, respectively, indicate measurement on heating and cooling.TCdetermined from the heating curves increases systematically with anneal time, implying that cation ordering occurs continuously and homogeneously at these temperatures. Cooling curves are virtually identical in all cases, showing that disordered states reached by re-equilibration atT>450 °C are quenched in at the cooling rate of theχ(T) experiment (~10 °C min−1). Note that NV39-A also has a (mostly) reversibleTCat ~580 °C associated with oxyexsolved, magnetite-rich grains. Figure 3: Curie temperature variation with anneal time. ( a ) Temperature-dependent susceptibility measurements and ( b ) derivative curves from samples MSH002-G following annealing at 350 °C for different durations. ( c , d ) Same data for NV39-A following annealing at 400 °C for different durations. Solid and dashed lines, respectively, indicate measurement on heating and cooling. T C determined from the heating curves increases systematically with anneal time, implying that cation ordering occurs continuously and homogeneously at these temperatures. Cooling curves are virtually identical in all cases, showing that disordered states reached by re-equilibration at T >450 °C are quenched in at the cooling rate of the χ ( T ) experiment (~10 °C min −1 ). Note that NV39-A also has a (mostly) reversible T C at ~580 °C associated with oxyexsolved, magnetite-rich grains. Full size image The same general behaviour was found in all specimens studied from both MSH ( Fig. 4a ) and NV ( Fig. 4c ); T C,heating increases systematically with both increased anneal time and anneal temperature, while T C, cooling remains nearly constant. To compare specimens that have slight but systematic differences in T C , we calculate the difference between the T C values determined from the heating and cooling legs (Δ T C ), which is approximately linear with ln(t) for all specimens ( Fig. 4b ). It is important to note that this behaviour is completely reproducible and ‘reversible’; Curie temperatures are decreased in thermomagnetic runs with T max >500 °C, and increased again by isothermal annealing at 350 or 400 °C, and the sequence can be repeated over and over without any significant permanent alteration. The exact same specimens were used for all anneal treatments, which were not carried out in direct order of increasing anneal time ( Supplementary Table S3 ). The systematic increase in T C therefore cannot be due to any cumulative thermally induced changes in the chemical composition or crystal structure of the titanomagnetites. 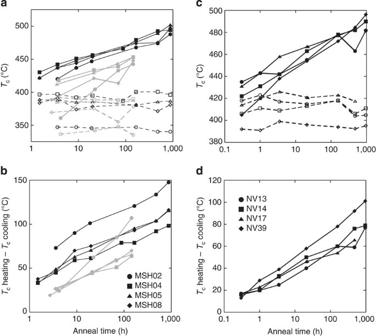Figure 4: Time- and temperature-dependent evolution of cation ordering. Cation ordering evolution inferred from Curie temperature in natural titanomagnetites from four MSH sites (a,b) and four NV sites (c,d). Samples annealed for variable durations at 400 °C (black symbols) and 350 °C (grey symbols). (a,c)TCmeasured on heating (solid symbols/lines) and on cooling (open symbols/dashed lines) following each anneal. (b,d) Difference betweenTCmeasured on warming and on cooling (ΔTC) represents the relative change in order degree. The initial state before each annealing treatment is relatively disordered, resulting from a previousχ(T) run to 600 °C with a heating/cooling rate of 10 °C min−1.TCduring heating increases systematically with anneal temperature and time, approximately as log(t) for the range studied.TCdetermined for the cooling leg of theχ(T) runs shows no systematic variation with anneal temperature or time, but does differ significantly for the different samples, showing a moderate correlation with Mg and Ti content. Figure 4: Time- and temperature-dependent evolution of cation ordering. Cation ordering evolution inferred from Curie temperature in natural titanomagnetites from four MSH sites ( a , b ) and four NV sites ( c , d ). Samples annealed for variable durations at 400 °C (black symbols) and 350 °C (grey symbols). ( a , c ) T C measured on heating (solid symbols/lines) and on cooling (open symbols/dashed lines) following each anneal. ( b , d ) Difference between T C measured on warming and on cooling (Δ T C ) represents the relative change in order degree. The initial state before each annealing treatment is relatively disordered, resulting from a previous χ ( T ) run to 600 °C with a heating/cooling rate of 10 °C min −1 . T C during heating increases systematically with anneal temperature and time, approximately as log(t) for the range studied. T C determined for the cooling leg of the χ ( T ) runs shows no systematic variation with anneal temperature or time, but does differ significantly for the different samples, showing a moderate correlation with Mg and Ti content. Full size image Mössbauer results Room-temperature Mössbauer spectra also show significant changes before and after isothermal annealing. The most significant difference in the spectra is in the distributions of magnetic hyperfine fields (B HF ) for both the A and B subspectra, which show larger maximum values and narrower peaks after annealing ( Fig. 5 , Supplementary Table S4 ). 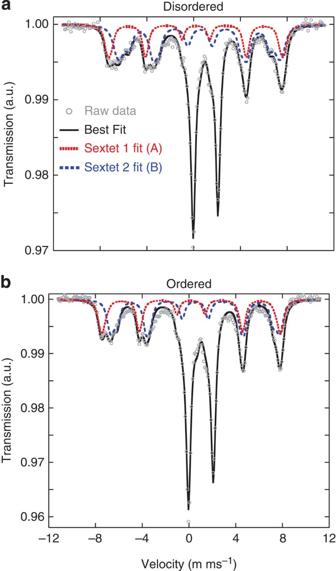Figure 5: Room-temperature ambient-field Mössbauer spectra. Sample MSH02-G in (a) a relatively disordered state (TC=337 °C) following rapid cooling from 600 °C, and (b) a relatively ordered state (TC=417 °C) produced by annealing at 350 °C for 114 h. The raw data are fit with two sextets to represent the ferromagnetic contribution from the titanomagnetite. For clarity, the two central doublet fits (paramagnetic Fe2+and Fe3+) are not shown. The A sextet effectively represents the tetrahedral Fe3+, while the B sextet represents the octahedral (and tetrahedral) Fe2.5+(seeSupplementary Methods). Figure 5: Room-temperature ambient-field Mössbauer spectra. Sample MSH02-G in ( a ) a relatively disordered state ( T C =337 °C) following rapid cooling from 600 °C, and ( b ) a relatively ordered state ( T C =417 °C) produced by annealing at 350 °C for 114 h. The raw data are fit with two sextets to represent the ferromagnetic contribution from the titanomagnetite. For clarity, the two central doublet fits (paramagnetic Fe 2+ and Fe 3+ ) are not shown. The A sextet effectively represents the tetrahedral Fe 3+ , while the B sextet represents the octahedral (and tetrahedral) Fe 2.5+ (see Supplementary Methods ). Full size image We interpret the observed changes in T C during thermomagnetic experiments and after isothermal annealing to be associated only with the homogeneous titanomagnetite grains. When present, the higher (>550 °C) T C consistent with magnetite-rich oxyexsolved grains remains unaffected by annealing or by thermomagnetic analysis. Several mechanisms may therefore be considered as possible causes of the observed changes in T C during thermomagnetic experiments and after isothermal annealing: oxidation/reduction; exsolution/rehomogenization; and cation disordering/reordering. Careful consideration of each will show that the former two are highly unlikely to account for our observations and that the third is the best available explanation. It has long been known that single-phase oxidation increases the T C of titanomagnetites. For high degrees of titanomaghemitization, T C is increased relative to the unoxidized stoichiometric state by amounts comparable to the changes that we have observed [26] , [27] . This might conceivably account for the observed increase in T C during annealing in air, although it seems improbable that oxidation would occur homogeneously and progressively throughout the volume of the titanomagnetites. Moreover, it is inconceivable that the reverse process would occur during the χ ( T ) runs in air, reducing highly oxidized titanomaghemite to stoichiometric titanomagnetite within minutes at 500 °C. Alternating exsolution and homogenization of the grains are also an implausible explanation. There are two processes by which this may occur: subsolvus unmixing into end-member magnetite and ulvöspinel, and oxyexsolution of ilmenite lamellae in a matrix of relatively pure magnetite. Oxyexsolution and rehomogenization can be ruled out for the same reason as homogeneous oxidation/reduction: χ ( T ) treatments in air could not reverse any previous oxidation. End-member unmixing is perhaps suggested by thermodynamically calculated solvus curves, which show that homogeneous titanomagnetite with compositions near x =0.3 or 0.4 become unstable at temperatures below about 400–500 °C (for example, ref. 28 ). However, the solvus curves are calculated for pure titanomagnetite, and experimental evidence suggests that the solvus is shifted to higher temperatures by the inclusion of Mg and Al [29] . Rehomogenization at 500 °C thus seems unlikely, especially on timescales of minutes. Compared with cation redistribution on sub unit cell scales, the kinetics of cation diffusion over length scales of many unit cells must be much slower [18] . Further, unmixing either by spinodal decomposition or by nucleation and growth would not be expected to produce the observed homogeneous, single-phase changes. We are therefore led to interpret the experimental results in terms of time- and temperature-dependent cation ordering in the titanomagnetites. As T C reflects exchange coupling between Fe 2+ and Fe 3+ (as well as cations of Mn or Cr, when present), the distribution of these cations between the magnetic sublattices will have a strong effect on T C . This is predicted by a Landau thermodynamic model [30] and has been well documented in magnesioferrite (MgFe 2 O 4 ), for which T C varies by ~70 °C between a state of relatively high order (equilibrated at 500 °C) and a strongly disordered state (equilibrated at 1,000 °C) [14] , [31] . Given sufficient time to equilibrate, the cation distribution will be more ordered at lower temperatures, with correspondingly higher Curie temperatures ( Fig. 6a ). However, our data are best explained by a system that is not in equilibrium at temperatures below ~450 °C. Initially disordered samples annealed isothermally at T <450 °C all show a progressive increase in T C with increasing anneal time, demonstrating that they are becoming progressively more ordered, but have not yet reached equilibrium, even after 10 3 h at 400 °C (for example, Fig. 6b ). In contrast, disordering occurs relatively rapidly at higher temperatures (>~450 °C) during the χ ( T ) experiments, and the relatively high degree of equilibrium disorder obtained at T >450 °C is quenched in by cooling to lower temperatures, resulting in a lower T C measured on cooling ( Fig. 6b ). That higher Curie temperatures (associated with greater order) are achieved on annealing at 400 °C compared with 350 °C is not reflective of an equilibrium condition, but demonstrates that the kinetics of the reordering are more rapid at 400 °C. 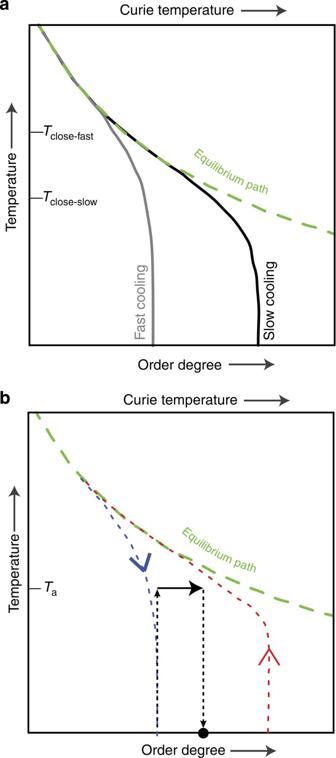Figure 6: Schematic representation of equilibrium order degree versus temperature. Dashed green line is equilibrium curve. (a) A rapidly cooled sample will follow the grey curve, departing from equilibrium at relatively high temperature (at the rate-dependentTclose) and quenching in a low degree of order. A slowly cooled sample will follow the black curve, departing from equilibrium at a lower temperature and quenching in a higher degree of order. (b) Duringχ(T) measurements, a sample cooled slowly in nature may follow the red path on heating and the blue path on cooling, resulting in a large thermomagnetic irreversibility. If this same sample is then subjected to annealing in the lab at temperatureTa, it will rapidly follow the black dashed line toTa, then slowly follow the solid black arrow during isothermal annealing. Upon quench, it will rapidly follow the black dashed line, ending at the solid black dot. Ifχ(T) is then measured on this same sample, the order degree would start at the black dot and follow a path towards the equilibrium curve. On cooling, it would again follow the blue dashed line. Figure 6: Schematic representation of equilibrium order degree versus temperature. Dashed green line is equilibrium curve. ( a ) A rapidly cooled sample will follow the grey curve, departing from equilibrium at relatively high temperature (at the rate-dependent T close ) and quenching in a low degree of order. A slowly cooled sample will follow the black curve, departing from equilibrium at a lower temperature and quenching in a higher degree of order. ( b ) During χ ( T ) measurements, a sample cooled slowly in nature may follow the red path on heating and the blue path on cooling, resulting in a large thermomagnetic irreversibility. If this same sample is then subjected to annealing in the lab at temperature T a , it will rapidly follow the black dashed line to T a , then slowly follow the solid black arrow during isothermal annealing. Upon quench, it will rapidly follow the black dashed line, ending at the solid black dot. If χ ( T ) is then measured on this same sample, the order degree would start at the black dot and follow a path towards the equilibrium curve. On cooling, it would again follow the blue dashed line. Full size image It is surprising to observe such large effects in these natural samples (Δ T C up to ~150 °C) given that previous studies have found either little or no evidence of temperature-dependent cation ordering in titanomagnetites [3] , [8] , [12] or relatively small changes in T C (Δ T C <40 °C) arising from cation reordering [15] . The small amount of Mg and Al substitution in these titanomagnetites may have a role in the effect, but we note that a study of similarly impure synthetic titanomagnetites (Fe 2.6 Ti 0.2 Mg 0.2 O 4 ) also found no evidence for temperature-dependent cation ordering [8] . One key difference between earlier studies and the present study is the temperature interval investigated. In previous studies, samples were annealed at and quenched from a range of temperatures >600 °C (refs 3 , 8 , 12 ). At these temperatures, the kinetics of the ordering process are likely fast enough that significant reordering occurs during quenching. This is suggested by the stepwise χ ( T ) experiment ( Fig. 2 ), which shows that once the specimen is heated to T >500 °C, T C remains constant at ~345 °C, regardless of the maximum temperature attained in subsequent heating/cooling cycles. For T >~500 °C, the cation ordering process achieves equilibrium at rates faster than the cooling rate of the χ ( T ) experiment (10 °C min −1 ) and remains on the temperature-dependent equilibrium path ( Fig. 6 ). The temperature at which the sample departs from the equilibrium path on cooling has been called the ‘closure temperature’ [18] . This closure temperature is rate dependent, and quenching at a fixed rate from any T > T close results in the same degree of observed order at room temperature. In Fig. 6a , for example, any sample cooled at the same ‘fast’ rate from T > T close-fast will end with the same order degree, because for all T > T close-fast the cation distribution remains on the equilibrium path. Only when samples are annealed at and quenched from T < T close (as in our experiments) will variations in ordering be observed. This interpretation of temperature-dependent cation ordering is supported by the Mössbauer spectroscopy data ( Fig. 5 , Supplementary Table S4 ). After rapid cooling from 600 °C, the broadened absorption peaks can be explained by chemical/structural disorder and variable local symmetry around the ferrous and ferric ions. Such an effect is predicted by Banerjee et al . [19] , who note that a more ordered cation distribution produced by slow cooling should produce narrower B sextet peaks. There is also an apparent change in the area ratio of the octahedral (B) and tetrahedral sites (A), with B/A being larger in the more disordered state. Although there is considerable uncertainty in the interpretation of area ratios for natural titanomagnetites, this observation appears to be consistent with the interpreted change in cation ordering ( Supplementary Methods ). One of the more interesting aspects of our experimental results is the lack of observed variation in room-temperature susceptibility or M S , combined with very large variations in T C . According to O’Reilly [32] , the cation distribution should have strong effects on M S and relatively weak control over T C , although the latter is typically underestimated (see below). To evaluate the potential effect of cation ordering on M S and T C , we may write a generalized structural formula allowing varying degrees of Fe cation ordering [11] , [12] as Fe 3+ b Fe 2+ 1− b [Fe 2+ b + x Fe 3+ 2−2 x − b Ti 4+ x ]O 4 , where 0≤ x ≤0.5 and the inversion parameter b ranges from 0 (normal spinel with no tetrahedral Fe 3+ ) to 1 (inverse spinel with only Fe 3+ in the tetrahedral site). Intermediate values of b correspond to disordered states with mixed-valence Fe cations on both sites, and for b =2/3 the distribution is random. For a composition of x ~0.3, as we have in our natural samples, the Weiss molecular field theory model of Stephenson [33] predicts a range of Curie temperatures from 408 °C for the most ordered arrangement ( b =1) to 343 °C for the random arrangement ( b =2/3). This calculated range is significantly smaller than the range that we have found experimentally. Further experimental evidence from synthetic titanomagnetites [15] and from synthetic magnesioferrites [14] , [18] suggests that the Stephenson [33] model substantially underestimates the effects of cation ordering on T C , probably due to associated effects including cation vacancies [15] and the interaction of magnetic ordering and cation ordering [14] , [18] . According to the same generalized structural formula, with atomic moments of 4 and 5 Bohr magnetons (μ B ) for Fe 2+ and Fe 3+ , respectively, the net spontaneous magnetization at 0 K is 6(1− x )−2 b μ B per formula unit (pfu), assuming collinear A–B coupling. For the same composition ( x ~0.3), there is a difference of about 23% between the saturation magnetization of the fully ordered inverse spinel distribution ( b =1, M S = 2.20 μ B pfu) and that of the fully disordered cation distribution ( b =2/3, M S = 2.87 μ B pfu). We clearly should not expect either the fully ordered or fully random states to be attained in our experiments, but we find essentially no detectable difference in the saturation magnetization of our samples produced by thermal treatments, despite the large changes in T C that we believe are due to changes in degree of cation ordering. This is true for M S both at room temperature and at 10 K ( Supplementary Methods and Supplementary Fig. S1 ). This seeming contradiction can only be fully resolved in future studies aimed specifically at constraining the exact cation distribution. The question is how to arrange the cations in such a way that the net moment of the two sublattices combined remains nearly constant, even while the interactions between or within the sublattices have changed. When we allow Mg 2+ , Al 3+ and other cations (and perhaps a small fraction of vacancies) into the lattice, the number of possible arrangements in the A and B sites grows rapidly, and the ordered arrangement (which remains imperfectly known even when only Fe 2+ , Fe 3+ and Ti 4+ ions are involved) is very uncertain when substituted cations are present in significant amounts [34] . Recent work [22] has confirmed that Ti 4+ almost always goes into the octahedral site [12] when it is the only non-Fe cation, but it is well known that Mg 2+ will partition into either site [31] . Although Al 3+ has a relatively strong preference for the octahedral site, it is not uncommon to find it in the tetrahedral site, and even less is known about site preference or valence state of Mn [35] . Site vacancies add another layer of uncertainty to the problem, though Wanamaker and Moskowitz [11] have shown and Lattard et al . [15] have confirmed that higher numbers of cation vacancies appear to result in a more disordered cation distribution. It therefore remains an important problem to work out the details of the cation arrangements in the more ordered states achieved by annealing, for which exchange interactions are strengthened enough to raise the T C by at least 150 °C, but in which the net moment differs little from that of the more disordered state achieved by rapid cooling. The common composition of the titanomagnetites studied here ( Fig. 1 ) suggests that the observed thermomagnetic effects could be important in a wide variety of natural materials. Exploitation of the cation ordering effect should allow us to constrain thermal histories of titanomagnetite-bearing rocks for T < T closure . Similar geospeedometers have been developed for orthopyroxene [36] and other silicates [37] , [38] , [39] , but the advantage of using titanomagnetite is that T C is an easily measured proxy for cation ordering, whereas in the silicate systems, ordering must be measured by more complicated means such as X-ray or neutron diffraction. Our findings have important implications for the interpretation of rock magnetic and paleomagnetic data, and irreversible thermomagnetic behaviour similar to that observed here ( T C ,heating > T C ,cooling ) is not uncommon in the literature [40] , [41] , [42] . It is typically attributed to chemical alteration or is not discussed, and T C is frequently taken to be an intrinsic property directly linked to Ti content. Even in pure titanomagnetites in the Fe-Ti-O system, some scatter in the relationship between T C and composition ( x ) is observed in experimental data (see review by Lattard et al . [15] ). For example, at x =0.4, the spread in T C of ~55 °C corresponds to approximately ±0.05 uncertainty in x , based on a polynomial fit to all available data. Explanations for this scatter have included heterogeneity or uncertainty in composition [6] , [15] or stoichiometry [6] , [11] , [43] ; thermomagnetic measurement methodology [15] ; or cation distribution [11] , [15] . The data presented here demonstrate that the uncertainty in using T C to determine composition is much greater, at least in the case of most natural samples that contain some degree of Mg and Al substitution. Another practical consideration is the impact of paleomagnetic thermal treatments on magnetic behaviour. Significant inferred changes in cation ordering occur in these samples and in some synthetic titanomagnetites [15] at temperatures just above and even below T C , in contrast to those in magnesioferrites [14] , [18] , where substantial ordering and disordering occur only at T >> T C . Routine thermal treatments in paleomagnetic or paleointensity studies will cause significant changes in the thermomagnetic behaviour of samples like these, and these changes may be impossible to recognize by monitoring room-temperature susceptibility. More fundamentally, our findings have major implications for theoretical models of thermoremanence, which remain firmly rooted in the thermal relaxation theory of Néel [7] for single-domain grains. It is a basic assumption of this theory that T C is a material constant, depending only on chemical composition and crystal structure of the remanence-carrying minerals, and that the function M S ( T ) is a single-valued and invariant material property, governing not only magnetization intensities but also the scaling of temperature-dependent anisotropies and energy-barrier distributions [44] , [45] , [46] , [47] , [48] , [49] , [50] , [51] , [52] , [53] . When the T C is itself a function of thermal history, and when M S ( T ) depends on the time- and temperature-dependent degree of cation ordering, additional complexity is required in quantitative modelling of remanence blocking and unblocking. In conclusion, we demonstrate here that T C in a set of natural titanomagnetites is strongly influenced by prior thermal history. Large (up to 150 °C) and reversible changes in T C are produced by annealing for 10 −1 to 10 3 h at 350–400 °C. We interpret these variations in T C to arise from temperature-dependent cation reordering, and Mössbauer spectroscopy data are consistent with this interpretation. As this reordering can occur during annealing (or slow cooling) at temperatures just above or below T C , the findings have important implications for our theoretical understanding of thermoremanence acquisition. Practically, the common composition of these natural titanomagnetites means that similar behaviour may have an important role in paleomagnetic studies of many natural rocks. Electron microprobe measurements Electron microprobe measurements were made on a JEOL JXA-8900 Electron Probe Microanalyser at the University of Minnesota. Cations measured were Fe, Ti, Mg, Al, Mn and Cr. Probe conditions included an accelerating voltage of 15 keV and a 15-nA beam current. Fe, Ti and Mn were calibrated on Smithsonian standard ilmenite USNM 96189, and Cr, Al and Mg were calibrated on Smithsonian standard magnesiochromite USNM 117075 (ref. 54 ). Measurements were made on magnetic extracts to increase the number of crystals that could be analysed in a single session. Analysed crystals were all homogenous phenocrysts with no visible reaction or exsolution features. Thermomagnetic measurements Initial magnetic characterization of the samples included single-cycle or multicycle thermomagnetic measurements, either low-field AC susceptibility ( χ ( T ) measured on an AGICO KLY2 bridge with CS2 furnace and temperature controller) or strong-field direct current magnetization ( M S ( T ) measured on a Princeton Measurements Corporation 3900 vibrating-sample magnetometer (VSM) with a flowing-helium furnace or on a horizontal Curie balance in air). χ ( T ) measurements were made at 10 °C min −1 , M S ( T ) at 10 °C min −1 (VSM) or 20 °C min −1 (Curie balance). Peak temperatures T max for the single-cycle runs were usually 600 or 650 °C, and when irreversible results were obtained, stepwise multicycle runs were done to constrain the temperature range associated with the irreversible behaviour. The stepwise experiments involved a set of heating/cooling cycles with increases in T max for each cycle, usually in increments of 50 or 100 °C. Curie temperatures were calculated from both the warming and cooling curves by finding inflection points of the χ ( T ) or M S ( T ) curves, where the downward curvature of the ferrimagnetic state gives way to the upward curvature of the paramagnetic state [55] , [56] . In practice this was done by finding the temperature for which the first derivative of the (three-point moving average) curve has a minimum (that is, greatest negative) value. For all data reported here, χ ( T ) measurements were made in air on bulk samples. However, based on tests with multiple samples, identical results are obtained for measurements made in argon and for magnetic separates. Mössbauer spectroscopy Resonant absorption of γ-rays by 57 Fe nuclei in a crystalline solid is sensitive to valence state, site coordination and magnetic ordering, and Mössbauer spectroscopy is therefore useful for examining the cation distribution in titanomagnetites [21] . We measured Mössbauer spectra at room temperature and in zero applied field for one specimen (MSH002-G-bn), prepared by pressing a magnetic extract with powdered boron nitride to produce a 25.4-mm-diameter, ~1-mm-thick disk that could be annealed and measured repeatedly. The sample was measured in two different states: after relatively rapid cooling (~60°C min −1 ) from 600 °C, and after heating at 350 °C for 114 h. See also Supplementary Methods . How to cite this article: Bowles, J. A. et al . Inferred time- and temperature-dependent cation ordering in natural titanomagnetites. Nat. Commun. 4:1916 doi: 10.1038/ncomms2938 (2013).